Two-colour pump–probe experiments with a twin-pulse-seed extreme ultraviolet free-electron laser Exploring the dynamics of matter driven to extreme non-equilibrium states by an intense ultrashort X-ray pulse is becoming reality, thanks to the advent of free-electron laser technology that allows development of different schemes for probing the response at variable time delay with a second pulse. Here we report the generation of two-colour extreme ultraviolet pulses of controlled wavelengths, intensity and timing by seeding of high-gain harmonic generation free-electron laser with multiple independent laser pulses. The potential of this new scheme is demonstrated by the time evolution of a titanium-grating diffraction pattern, tuning the two coherent pulses to the titanium M-resonance and varying their intensities. This reveals that an intense pulse induces abrupt pattern changes on a time scale shorter than hydrodynamic expansion and ablation. This result exemplifies the essential capabilities of the jitter-free multiple-colour free-electron laser pulse sequences to study evolving states of matter with element sensitivity. The rapid development of table-top high harmonic generation and free-electron laser (FEL) technologies generating coherent, intense and ultrashort extreme ultraviolet (XUV)/soft X-ray pulses is opening new frontiers of ultrafast science, pushing nonlinear optics into the X-ray domain and providing a basis for a variety of novel time-resolved schemes. Pump–probe techniques, first applied using optical lasers for studying non-equilibrium transient states of matter [1] , [2] , [3] , have now been extended to high harmonic generation- [4] , [5] , [6] and FEL- [7] , [8] , [9] , [10] generated pulses using either X-ray or synchronized optical and X-ray pulses pairs. The great advantage of XUV/X-ray photons is that they can stimulate and probe electronic transitions from core levels, providing chemical selectivity as well. Ultrabright FELs overcome the pulse intensity and wavelength tunability limitations of high harmonic generation sources, allowing experiments not possible a few years ago. Among the numerous exciting opportunities are studies of exotic properties of matter driven into non-equilibrium transient states by ultrabright X-ray pulses [11] , [12] , [13] , [14] ; these studies are relevant to inertial fusion [15] , planetary interior physics [16] and, more generally, to radiation–matter interactions [17] . To date, FEL pump–FEL probe schemes have been based either on time-delayed holography, where the ‘probe’ pulse is the ‘pump’ one returned by a mirror [18] , or on autocorrelator devices [19] , [20] . Both approaches give access only to single-colour experiments. Very recently, the LCLS group has reported [21] generating a pair of temporally and spectrally separate soft X-ray FEL pulses via a double undulator scheme. However, due to the underlying self-amplified spontaneous emission configuration, these pulses have partial longitudinal coherence and limited shot-to-shot repeatability in both energy and central wavelength. Here we report the successful generation, via two-colour, two-pulse external laser seeding of a high-gain harmonic-generation (HGHG)-based FEL, of two FEL pulses with precisely controlled time delay, wavelength and intensity ratio. These highly transversely and longitudinally coherent FEL pulse pairs are used in a proof-of-principle XUV pump–XUV probe experiment that examines the dynamics of a thin-metal layer structure exposed to high-intensity XUV excitation. Generation of twin FEL pulse The process leading to the generation of ultrafast XUV/X-ray light pulses in a HGHG FEL [22] , [23] begins with an external optical laser (seed). If the seed radiation spectrum is contained inside the gain bandwidth of the FEL amplifier and the amplification process does not enter into the deep saturation regime, the output radiation properties (spectrum, duration and arrival time) are very tightly correlated with those of the input seed laser pulse. This scheme is presently adopted at FERMI@Elettra and has demonstrated outstanding performances in terms of stability [10] , wavelength and polarization tunability [24] . As envisioned by Freund and O’Shea [25] , a straightforward method for the generation of multiple X-ray pulses from an HGHG FEL consists of seeding the electron bunch with multiple laser pulses. In the specific configuration demonstrated here, we use two ultraviolet, 180-fs duration (full-width at half-maximum) seed pulses at slightly different central wavelengths and (independently tunable in the 260–262 nm range) with variable time separation and intensity ratio. As schematically shown in Fig. 1a , these pulses are focused in the modulator undulator stage of the HGHG FEL and interact with a mildly compressed 750-fs-long electron bunch, for which particular attention was devoted to preserve the temporal uniformity of the beam parameters (mainly current and energy; see Supplementary Fig. S1 and Supplementary Note 1 ). A fourth harmonic (that is, X-band) radiofrequency cavity installed before the magnetic chicane linearizes the longitudinal phase space of the electron beam to obtain a nominally flat current (~500–600 A). It was operated close to the maximum decelerating phase at a gradient of about 17 MV m −1 and compensates both for nonlinear E ( t ) terms due to the radiofrequency curvature of the upstream accelerator sections and for the second-order momentum compaction term of the chicane itself. 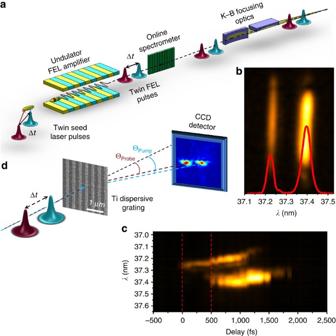Figure 1: Generation and characterization of the twin-seeded FEL pulses and experimental set-up. (a) Energetically distinct two ultraviolet laser pulses with an adjustable delay interact with a single electron bunch. Inside the FEL amplifier, the two seeded regions emit XUV radiation. The wavelength and temporal separation of generated twin FEL pulses are determined by the parameters of the seed laser pulses and the spectral purity, pulse intensities and widths of the pulses is monitored by an ‘online’ spectrometer. (b) Typical spectrum of the twin-FEL pulses. (c) Sequence of FEL spectra obtained during a temporal scan of the seed laser pulse pair with respect to the electron bunch. The zero time is defined as the instant when the first laser pulse interacts with the electron bunch. Increasing the arrival time delay of the laser pulses with respect to the electron bunch, the emission of the second FEL pulse is evident after ~500 fs. The relative time separation, marked by the dashed red line, between the two FEL spectral lines ensures that the temporal structure of the twin FEL emission is determined by the delay between the seed laser pair. (d) Experimental layout: the twin FEL pulses with different wavelength, focused by K–B optics (shown in (a)), impinge on the Ti grating (80-nm thick and 165-nm wide Ti strips with 400-nm pitch fabricated on a 20-nm thick Si3N4window) and are diffracted along the horizontal plane. The seventh order diffraction pattern is detected by a CCD camera placed off-axis with respect to the direct beam. Figure 1: Generation and characterization of the twin-seeded FEL pulses and experimental set-up. ( a ) Energetically distinct two ultraviolet laser pulses with an adjustable delay interact with a single electron bunch. Inside the FEL amplifier, the two seeded regions emit XUV radiation. The wavelength and temporal separation of generated twin FEL pulses are determined by the parameters of the seed laser pulses and the spectral purity, pulse intensities and widths of the pulses is monitored by an ‘online’ spectrometer. ( b ) Typical spectrum of the twin-FEL pulses. ( c ) Sequence of FEL spectra obtained during a temporal scan of the seed laser pulse pair with respect to the electron bunch. The zero time is defined as the instant when the first laser pulse interacts with the electron bunch. Increasing the arrival time delay of the laser pulses with respect to the electron bunch, the emission of the second FEL pulse is evident after ~500 fs. The relative time separation, marked by the dashed red line, between the two FEL spectral lines ensures that the temporal structure of the twin FEL emission is determined by the delay between the seed laser pair. ( d ) Experimental layout: the twin FEL pulses with different wavelength, focused by K–B optics (shown in ( a )), impinge on the Ti grating (80-nm thick and 165-nm wide Ti strips with 400-nm pitch fabricated on a 20-nm thick Si 3 N 4 window) and are diffracted along the horizontal plane. The seventh order diffraction pattern is detected by a CCD camera placed off-axis with respect to the direct beam. Full size image After final acceleration to 1.2 GeV, the electron beam is first energy-modulated by the seed pulses in a short undulator and, afterwards, passage through a chromatic dispersion section leads to the formation of two density-modulated regions in which the phase/amplitude properties of the two seed pulses are encoded into the electrons. In the final radiator undulator sections, whose magnetic strengths ( K ) are tuned for fundamental FEL resonance with the N th harmonic ( N =7 in our case) of the average seed wavelength, these two regions emit two temporally and spectrally independent XUV pulses at and , whose relative delay can be controlled by tuning the delay between the input seed pulses. Although the seed laser is linearly polarized, the FERMI undulators have variable polarization, permitting choice of either linear or helical output polarization. Among the different possible schemes to generate two-colour, ultraviolet-wavelength, fs-duration seeding laser pulses, we chose the following as best matched to our particular seed laser system and pump–probe experiment. Given the goal of producing two cleanly separated ultraviolet output pulses with slightly different wavelengths, we introduced the seed pulse splitting already at the fundamental wavelength (784 nm). The 120-fs long infrared pulses were divided into two parallel, independent channels for third harmonic generation (THG). Each channel consists of a type 1, second harmonic generation beta-barium borate crystal, a birefringent delay plate, a polarization rotator that rotates by 90° the polarization of the second harmonic light only and a type 1, THG beta-barium borate crystal mounted on a rotation stage. A pair of 4° fused silica wedges provides fine tuning (in the range from 0 to ±2.5 ps) of the delay of the ultraviolet pulse generated in one of the arms. In this experiment, the second harmonic generation/THG crystal length was chosen to generate pulses of duration in the range 180–200 fs. The central wavelength of both pulses can be independently tuned in the 260–262-nm range by crystal rotation in the main crystal axis plane (see Supplementary Fig. S2 ). The output ultraviolet pulses duration and separation were measured by a cross-correlator using as a reference a fraction of the pulses from the Ti:Sapphire oscillator that seed the amplifier section of the seed laser. As would be expected, cross-correlation traces taken both repetitively and over different time separations indicate the absence of any measurable timing jitter or drifts between the two generated ultraviolet pulses (see Supplementary Fig. S2 and Supplementary Note 2 ). The seed pulses were then transported and focused at the modulator undulator centre using the standard FERMI optical configuration [10] , [24] . After aligning the relative electron beam and seed timing, so that the FEL would lase only on the first pulse at (referred to as the ‘pump’), a fine scan of the relative seed/electron-beam timing ( Fig. 1c ) was performed in order to find an optimum position in the leading edge of the electron bunch. This ensures that a sufficiently wide, unused portion of electrons towards the tail could accommodate the second ultraviolet pulse (referred to as the ‘probe’). When both seed pulses were injected into the HGHG FEL, clean, twin peak output spectra were observed if the temporal delay between the two pulses was set in the proper range. The pump–probe delay for this experiment was between about 300 and 700 fs, limited on the upper side by the electron bunch length and on the lower one by the seed pulse duration. For shorter delays, interference effects lead to spectral modulation. Figure 1b shows a typical spectrometer image of the twin FEL pulses generated with a time delay of 500 fs. As can be seen from the figure (and from the Supplementary Movie 1 ), the spectrum in this twin-pulse seeded regime is extremely clean and stable. The performance of the twin-pulse-seeding scheme in terms of spectral purity and intensity stability compared with single-seed FEL emission is displayed in Fig. 2 . The results are obtained recording 1,150 consecutive spectra on both the ‘online’ spectrometer ( Fig. 2a ) and the total FEL intensity on the I 0 gas monitor detector [26] ( Fig. 2b ). The switching between the single and double FEL emissions is obtained by blocking one of the seed laser arms, without changing the electron-beam characteristics nor the undulator strength parameter K . Fitting the two-colour FEL spectra as a sum of two independent Gaussians, we estimate a negligible difference between the single and double FEL emissions, confirming the robustness of the pulse generation scheme. Statistical analysis of the spectra in Fig. 2a shows that the root mean square bandwidth is about 25 × 10 −3 nm, that is, ~0.05% of the central wavelength, together with a shot-to-shot peak position root mean square jitter of about 3 × 10 −3 nm (about 0.005% of the central wavelength, Fig. 2c ). 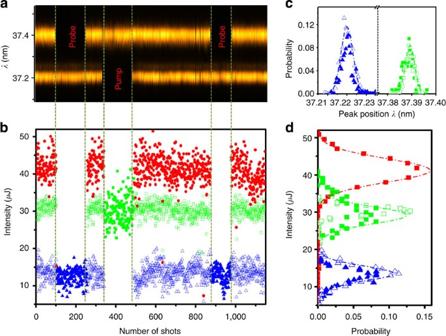Figure 2: Spectral and intensity stability of twin-seeded FEL radiation. Sequence of 1,150 consecutive single-shot FEL emission spectra (a) and corresponding intensities (b). Green dash lines highlight the intentional blocking of one of the seed laser arms (pump or probe) in order to suppress one of the FEL pulses. The filled markers identify the FEL emission configuration: double FEL emission using twin laser seed pulses (red circles, total signal), single FEL emission probe signal only (blue triangles) and single FEL emission pump signal only (green squares). The open markers are the absolute intensities of a single pulse (green for pump and blue for probe) for two-colour emission, obtained from the corresponding peak area in the spectra. Probability distribution for the peak wavelength jitter (c) and emission intensity (d). The colours correspond to the configurations reported in panel (b). Figure 2b shows that the absolute single-wavelength intensities of double FEL emission, obtained from the corresponding peak area of the spectrum (see Supplementary Fig. S3 and Supplementary Note 3 ), is comparable to those of single FEL emission, with a root mean square shot-to-shot stability of about 15% ( Fig. 2d ). In the adopted scheme, the intensity ratio between the pump and probe pulses can be tuned easily by changing the relative intensity of either seed laser pulse. This can also be accomplished by changing the normalized strength K of the FEL undulators to favour the growth of one of the pulses over the other. Figure 2: Spectral and intensity stability of twin-seeded FEL radiation. Sequence of 1,150 consecutive single-shot FEL emission spectra ( a ) and corresponding intensities ( b ). Green dash lines highlight the intentional blocking of one of the seed laser arms (pump or probe) in order to suppress one of the FEL pulses. The filled markers identify the FEL emission configuration: double FEL emission using twin laser seed pulses (red circles, total signal), single FEL emission probe signal only (blue triangles) and single FEL emission pump signal only (green squares). The open markers are the absolute intensities of a single pulse (green for pump and blue for probe) for two-colour emission, obtained from the corresponding peak area in the spectra. Probability distribution for the peak wavelength jitter ( c ) and emission intensity ( d ). The colours correspond to the configurations reported in panel ( b ). Full size image Proof-of-principle pump and probe experiment As the wavelengths of the twin pulses are rather close, we used a Ti grating ( Fig. 1d ) that acts as a spectral analyser, separating angularly the diffraction peaks of the pump and probe pulses. The wavelength and intensity of each pulse were measured by the I 0 gas monitor and the ‘online’ spectrometer ( Fig. 1a ). The maximum pulse intensity for the pump pulse was 30 μJ, corresponding to a fluence ( F ) of about 18.5 J cm −2 on the sample, and was attenuated using a gas cell and/or Al solid-state filters. The diffraction measurements were carried out at the DiProI end station [27] , where the FEL pulses were focused to a 195±30 μm 2 spot on the sample by a Kirkpatrick–Baez (K–B) active optical system [28] . As shown in Fig. 1d , the pulses hit the sample at normal incidence and diffract along directions defined by the transmission grating angles: , where λ 1,2 and N d are the FEL wavelengths and the diffraction order, respectively, and b is the grating pitch. The two-colour pulses were tuned to wavelengths in the slope region above the Ti M 2/3 edge ( λ ~38 nm). By tuning to an atomic resonance we become more sensible in terms of photon deflection angle and absorption, as the monotonic wavelength dependence of both dispersive ( δ ) and absorptive ( β ) terms of the complex refractive index undergoes sharp changes through the atomic resonances [29] . Consequently the diffraction peak intensities and positions are highly sensitive to the Ti ionization state at the arrival time of the probe pulse. Performing sets of measurements with different samples and varying the fluence, we determined that the ‘radiation damage’ threshold is around 150 mJ cm −2 (see Supplementary Figs S4–S5 and Supplementary Note 4 ). 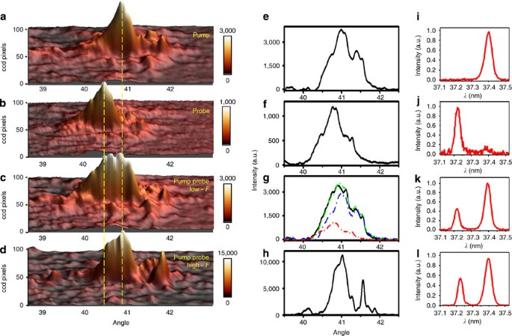Figure 3: Diffraction as a function of the FEL intensity. Diffraction patterns obtained usingλ1=37.39±0.03 nm (pump) andλ2=37.22±0.03 nm (probe) pulses with a pump–probe delay of 500 fs. (a) Single-colour low-Fpump (~32 mJ cm−2per pulse). (b) Single-colour low-Fprobe (~9 mJ cm−2per pulse). (c) Two-colour low-Fpump and probe (pump~31 mJ cm−2per pulse, probe~11 mJ cm−2per pulse). (d) Two-colour high-Fsingle-shot pump and probe (pump~2.5 J cm−2, probe~1.0 J cm−2). The low-Fpatterns ina–care obtained integrating over 150 shots. Yellow dash lines indicate the positions of diffraction peaks for the pump and probe pulses of the low-Funperturbed state. The panelse,fshow the diffraction line-shape along the dispersive direction of the Ti grating. Ingthe diffraction line profile of the pump–probe pattern (black line) is compared with the sum (dashed green line) of the pump (dashed blue line) and probe (dashed red line) profiles, weighted to the corresponding pulse intensity. The featured line-shape and the differences in the profiles of the pump and probe pulses are due to structural imperfections of the grating. The corresponding spectra of the incident beam are shown in the panelsi–l. Figure 3a–c show the results, representing the low- F regime ( F <150 mJ cm −2 ) when the radiation induces minor changes in Ti electronic structure. In this ‘unperturbed’ regime the diffraction patterns have the expected peak position and, more relevantly, the two-colour (pump–probe) pattern is a sum of the pump ( Fig. 3a ) and the probe ( Fig. 3b ) peaks. This is evidenced by the deconvolution of the pump–probe line profile shown on Fig. 3g in its two radiation components profile (that is, pump Fig. 3e and probe Fig. 3f ) weighted by their relative pulse intensity measured using the ‘online’ spectrometer ( Fig. 3i–k , see also Supplementary Note 3 ). Figure 3: Diffraction as a function of the FEL intensity. Diffraction patterns obtained using λ 1 =37.39±0.03 nm (pump) and λ 2 =37.22±0.03 nm (probe) pulses with a pump–probe delay of 500 fs. ( a ) Single-colour low- F pump (~32 mJ cm −2 per pulse). ( b ) Single-colour low- F probe (~9 mJ cm −2 per pulse). ( c ) Two-colour low- F pump and probe (pump~31 mJ cm −2 per pulse, probe~11 mJ cm −2 per pulse). ( d ) Two-colour high- F single-shot pump and probe (pump~2.5 J cm −2 , probe~1.0 J cm −2 ). The low- F patterns in a – c are obtained integrating over 150 shots. Yellow dash lines indicate the positions of diffraction peaks for the pump and probe pulses of the low- F unperturbed state. The panels e , f show the diffraction line-shape along the dispersive direction of the Ti grating. In g the diffraction line profile of the pump–probe pattern (black line) is compared with the sum (dashed green line) of the pump (dashed blue line) and probe (dashed red line) profiles, weighted to the corresponding pulse intensity. The featured line-shape and the differences in the profiles of the pump and probe pulses are due to structural imperfections of the grating. The corresponding spectra of the incident beam are shown in the panels i – l . Full size image Figure 3d shows the single-shot, pump–probe pattern for the high- F regime, which results in a diffraction pattern where the contribution of the probe peak appears strongly attenuated (see also Fig. 3h ). Since the duration of the experiment, considering that the estimated FEL pulse length (~90 fs) [10] and the delay (~500 fs) are shorter than the time scales of hydrodynamic expansion of 1–10 ps (refs 18 , 30 ), the two pulses probe practically the same grating geometry. We estimated that the expansion of the Ti grating line profile for these conditions is smaller than 2.5 nm. Consequently, the distinct difference in the Fig. 3c,d patterns indicates that the intense pump pulse induces dramatic changes in the Ti electronic structure. As already reported [31] , [32] , the high degree of ionization created by the pump shifts the absorption resonances to shorter wavelengths. For wavelengths tuned to the material absorption resonance such shift will induce abrupt changes in the complex index of refraction n =1– δ + i·β , resulting in a decrease of the diffracted peak intensity and width. The observed trend can be qualitatively understood in terms of the deposited energy during the pump pulse. In the low -F regime, <1% of Ti atoms are ionized by the pump. In this case the optical properties of the material are negligibly affected by the material ionization state. Conversely, at high -F , almost all Ti atoms are ionized within a few 10’s of fs. The generated primary photoelectrons then thermalize creating high ionization states through secondary electron emission and Auger decay. These events occur at time scales shorter than 100 fs (refs 31 , 33 ) and, as a result, the absorption edge (and hence the optical constants δ and β ) is shifted towards shorter wavelengths [32] , [34] . 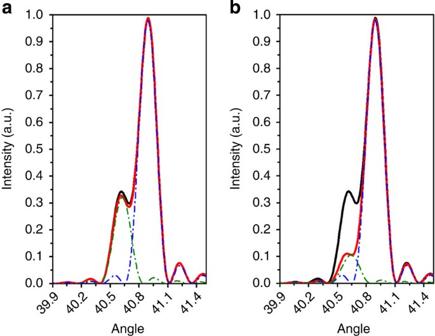Figure 4: Simulated diffraction line-shape. Calculated diffraction line-shape for the Ti grating illuminated by the two twin FEL pulses at 37.2 and 37.4 nm. Black lines are obtained by assuming no wavelength shift of the optical constant (that is, low-Fregime). Red lines panels (a,b) show the modification of the diffraction line-shape induced by 0.5- and 2.3-nm shift towards shorter wavelength of bothδandβfor the probe pulse. Blue and green dash-dot lines correspond to the diffracted signal from the pump and the probe, respectively. In the simulation, the same experimental ratio of 3:1 between the intensity of the pump and the probe was assumed. Figure 4 shows the calculated diffraction line-shape for the low -F (black line) and high -F (red line) regime, respectively. In the latter case, for the probe pulse, we assumed a rigid shift towards a shorter wavelength using the tabulated wavelength dependence of δ and β in ref. 29 , while no wavelength shift was considered for the pump. Figure 4: Simulated diffraction line-shape. Calculated diffraction line-shape for the Ti grating illuminated by the two twin FEL pulses at 37.2 and 37.4 nm. Black lines are obtained by assuming no wavelength shift of the optical constant (that is, low -F regime). Red lines panels ( a , b ) show the modification of the diffraction line-shape induced by 0.5- and 2.3-nm shift towards shorter wavelength of both δ and β for the probe pulse. Blue and green dash-dot lines correspond to the diffracted signal from the pump and the probe, respectively. In the simulation, the same experimental ratio of 3:1 between the intensity of the pump and the probe was assumed. Full size image Figure 4a shows that the experimental result cannot be reproduced for a small absorption edge shift of 0.5 nm (that is, when the probe wavelength remains within the absorption edge windows) ~500 fs after the pump excitation. A fair agreement with experiments requires assuming an absorption edge shift of 2.3 nm ( Fig. 4b ): in this case the probe signal (green dash dot line) is quenched. This trend is similar to the observed photo-induced transparency of Al [12] obtained by high-fluence FEL pulses and to the quenching of the X-ray resonant magnetic scattering signal on Co/Pt multilayer systems using very intense FEL pulses [34] . However, the approach reported here has the remarkable potential advantage of providing time resolution in the sub-ps domain to follow the FEL-induced changes in material electronic structure and non-thermal ion motions. We experimentally demonstrated the possibility to generate and use two distinct XUV FEL pulses with finely controllable wavelength and relative time delay by using a twin-pulse, external laser seeding of the HGHG-based FEL source (FERMI@Elettra). The FEL twin pulses used here had a relative time delay between 300 and 700 fs and central wavelengths of 37.2 and 37.4 nm, tuned to the Ti M 2,3 absorption edge. We exploited this newly developed tool to perform the first all-FEL-based, two-colour pump–probe experiment with specially designed Ti grating. For fluences >2 J cm −2 the obtained pump–probe diffraction patterns indicate the occurrence of a photo-induced transparency. This evidences the high degree of Ti ionization created by the intense pump pulse, which results in a sensible shift of the Ti absorption edge to wavelengths shorter than the probe one. This technique can easily be extended to generate pump–probe pulses with similar wavelength separation in the whole presently available FERMI-FEL1 range (65–20 nm). The possible extension of the reported technique to shorter wavelengths is naturally linked to the performance of the HGHG scheme at high harmonic orders. Although the limit of HGHG process at very high harmonics in a single-stage FEL can be overcome with a multistage approach [35] , the noise degradation in the frequency multiplication process [36] can prevent the implementation of this scheme at very short wavelength (few nm). However, single-stage HGHG process used in the FERMI-FEL1 amplifier has so far allowed a clear pulse generation at harmonic orders up to 22 (about 12 nm), so the double-pulse seed is expected to work fine in this spectral region. The minimum interpulse delay can be decreased to about 150 fs for the existing seed laser system. Shorter pulse delays comparable with the FEL pulse duration (we expect to reach 50–30 fs in the future) can be obtained by adopting another scheme that seeds with a single, frequency-chirped pulse and where deterministic spectro-temporal pulse-splitting occurs in the deep saturation regime of the FEL [37] , [38] . The current upper limit of delay between the two pulses can also be extended to above 1 ps by optimizing the FERMI photoinjector and linac in order to produce longer electron bunches with temporally flat output energy distributions. In the particular case reported here, the wavelength separation was limited to about 0.2 nm by the tuning bandwidth of the seed laser THG spectrum. This limitation can easily be overcome in the future by using the parametric amplifier as a source of one of the pulses which could then be tuned to any desired wavelength of the present seed ultraviolet tuning range (that is, 228–262 nm). The other pulse could still be generated by the THG channel at 261 nm. The main limitation then would come from the limited FEL gain bandwidth of the undulators, which is about 4–5% for the modulator and 0.5–1% for the radiator undulator chain. It should be noted that there are schemes overcoming also this limitation, for example, by introducing an energy/position correlation in the electron beam or, at some expense of the available output power, by selectively tuning the individual radiator resonances to the two seed wavelengths λ 1 / n and λ 2 / m . These configurations are under study for future developments. From a wider perspective, the concepts reported here for generating multiple and multi-colour coherent photon pulses with fully controllable parameters will open up the way to extend the most advanced, table-top ultrafast methods into the XUV/X-ray domain, thus potentially adding nanometre spatial resolution and atomic selectivity to these powerful experimental tools. This will advance our knowledge to the fundamental domains of materials science, paving the road to future nonlinear X-ray technologies that cannot even be foreseen today. K–B focusing optics The photons produced by the FEL source were focused on the sample plane by two bendable Au-coated (30 nm) planar mirrors placed in K–B configuration. The nominal focal length of the optical system is 1,750 mm for the vertical direction, and 1,200 mm for the horizontal one. The focal spot size, both in case of single- and double-emission FEL radiations, was optimized using a Hartmann wave front sensor detector placed at ~917 mm downstream to the FEL sample interaction region. FEL ablation of polymethyl methacrylate was used to determine spatial overlapping on the sample plane of the impinging radiation in the case of double emission FEL radiation. The spot size was estimated by back propagating the Hartmann wave front sensor wavefield to be 13 (±1) × 15(±1.5) μm 2 , in good agreement with the atomic force microscopy analysis of the craters produce by a single FEL shot on polymethyl methacrylate. Sample description The sample consists of Ti grating with 80-nm thick and 165-nm wide strips. The samples were fabricated by a combination of sputtering deposition, electron-beam lithographic and reactive ion etching processes on a 20-nm thick 50 × 50 μm 2 Si 3 N 4 window. A 5-nm Cr adhesion layer was deposited between Ti and Si 3 N 4 window and used as hard etching stopping mask in the reactive ion etching process. The pitch between the nano-lithographic lines is 400 nm and was controlled after the sample preparation with conventional electron-beam microscopy. Experimental set-up The diffraction pattern resulting from the interaction of the FEL pulses with the Ti grating was monitored on a Princeton Instrument PI-MTE back illuminated charged coupled device (CCD) camera with frame format 2048 × 2048 pixels and 13.5 μm pixels size. The CCD was mounted on X–Z translator stages that allow placing the detector at the correct grating diffraction angle. In the used experimental geometry the detector was positioned ~50 mm downstream the sample, off-axis by ~25 mm with respect to the FEL beam trajectory. Taking into account the sample layout, the experimental geometry and the wavelengths of the impinging FEL pulses ( λ 1 =37.2 nm and λ 2 =37.4 nm), the separation of the two Bragg spots (seventh order) on the CCD detector was ~27 pixels (that is, 4.5 mrad). How to cite this article: Allaria, E. et al. Two-colour pump–probe experiments with a twin-pulse-seed extreme ultraviolet free-electron laser. Nat. Commun. 4:2476 doi: 10.1038/ncomms3476 (2013).